Subfemtosecond steering of hydrocarbon deprotonation through superposition of vibrational modes Subfemtosecond control of the breaking and making of chemical bonds in polyatomic molecules is poised to open new pathways for the laser-driven synthesis of chemical products. The break-up of the C-H bond in hydrocarbons is an ubiquitous process during laser-induced dissociation. While the yield of the deprotonation of hydrocarbons has been successfully manipulated in recent studies, full control of the reaction would also require a directional control (that is, which C-H bond is broken). Here, we demonstrate steering of deprotonation from symmetric acetylene molecules on subfemtosecond timescales before the break-up of the molecular dication. On the basis of quantum mechanical calculations, the experimental results are interpreted in terms of a novel subfemtosecond control mechanism involving non-resonant excitation and superposition of vibrational degrees of freedom. This mechanism permits control over the directionality of chemical reactions via vibrational excitation on timescales defined by the subcycle evolution of the laser waveform. The nuclear kinematics that are responsible for making and breaking chemical bonds occur on femtosecond timescales [1] . The steering of chemical reactions has been demonstrated for a variety of systems in the gas and condensed phase using modulated light fields [2] , [3] , [4] , [5] , [6] , with the amplitude, phase and polarization used as a control parameter. Breaking of the hydrogen bonds is one of the most important dynamic reactions in the chemistry related to biology, combustion and catalysis, motivating considerable efforts to monitor and ultimately control the process. It has been studied in great detail, where efficient strong-field-induced proton ejection was reported [7] , [8] , [9] , [10] , [11] , [12] , [13] , [14] . Dynamic charge localization [11] and concerted fragmentation [12] scenarios were suggested to explain the origin of the high kinetic energies of the ejected protons. These studies corroborated the need for ultrashort light pulses, consisting of a few cycles, for steering the deprotonation process. As an additional challenge, the aforementioned control schemes do not provide means for a bond-specific manipulation of the deprotonation in symmetric hydrocarbons. Few-cycle pulses with well-defined waveforms [15] offer a new quality of control on direct manipulation of the wavefunction of a molecular system [16] . Few-cycle waveforms with adjustable carrier-envelope-phase (CEP) have permitted control of charge localization in the ionization and dissociation of diatomic molecules on a subfemtosecond timescale [17] , [18] , [19] , [20] , [21] . The approach has also been successful in altering the yields of ionization and fragmentation in hydrocarbons [13] . Despite its relevance to stereochemistry, that is, the rearrangements of atoms in a molecule, full control of the deprotonation of hydrocarbons, including the directional steering of the emission of the protons, has, however, not been reported. Here, we demonstrate the subfemtosecond control of the proton-ejection direction from acetylene molecules with the waveform of near-single-cycle laser pulses. On the basis of quantum dynamical calculations, we show that the demonstrated directional control does not originate from electronic motion effects considered so far [16] . Rather, the mechanism is based on the manipulation of the phases of individual components of the multi-mode vibrational wave packet by the laser field in the neutral molecule and cation. While control of vibrational superpositions and their phase after resonant excitation has been performed in the context of molecular vibrational qubits [22] , [23] , the superposition between vibrational modes is formed through a non-resonant process in our study and is controlled on an attosecond timescale. The process described here constitutes a novel mechanism for steering the reactions of complex molecules. Laser-induced deprotonation of the acetylene dication The electric field waveform of (transform-limited) few-cycle light pulses can be described as E ( t )= E 0 ( t ) cos( ωt + φ ), where E 0 ( t ) is the amplitude envelope, ω the carrier angular frequency and φ is the CEP. The CEP offers a way to tailor the electric field waveform on subfemtosecond timescales and has proven to be a powerful parameter for steering electron motion [16] . In our present experimental studies on the CEP control of the deprotonation of acetylene, we employ CEP-tagged reaction microscopy (REMI) [24] (for details see the Methods section). The interaction of acetylene molecules with intense few-cycle pulses results in the dissociative ionization and isomerization of the molecule yielding a variety of reaction products [7] . One of the reactions that we concentrate on here is the deprotonation of acetylene after two consecutive ionization steps, see Fig. 1a , where a 1D cut of the potential energy surfaces (PES) is shown. After population of the first excited state of C 2 H 2 2+ , the dication breaks up into H + and C 2 H + fragments, which are detected with the REMI in coincidence. 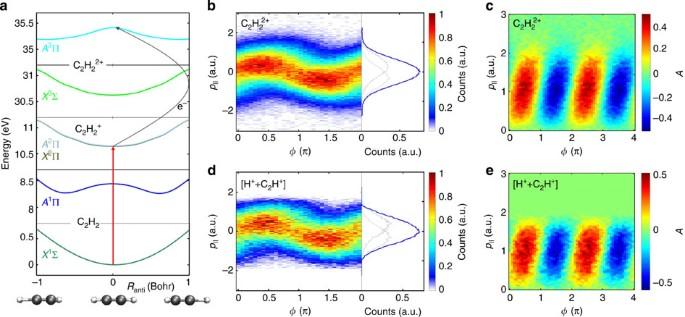Figure 1: Generation of the acetylene dication and the deprotonation fragments. (a) 1-D cut of potential energy curves of the considered states in the ionization and deprotonation: ground () and first excited state (A1Πu) of the neutral molecule, the cation ground (X2Πu) and degenerate first excited state (A2Πu), and the dication ground () and first excited state (A3Πu) along the anti-symmetric stretching coordinateRantiatRsym=0. The red vertical line indicates the tunnelling ionization and the grey curved line marks the second ionization step by electron recollision. (b) Density plot of the acetylene dication longitudinal recoil momentum as a function of the experimental CEP,φ, for 4 fs pulses at an intensity of 2 × 1014W cm−2. CEP-integrated momenta are shown in the right panel. The dashed (dotted) lines shown correspond to CEP’s with maximum positive (negative) asymmetry in the ion emission, respectively. (c) Density plot for the asymmetry parameter,A(p||,φ), for C2H22+ions. (d) Density plot of the vector momentum sum of the recoil of the two (H+,C2H+) deprotonation fragments. (e) Density plot of the asymmetry parameter for the momentum sum of the deprotonation fragments (H+,C2H+). Figure 1: Generation of the acetylene dication and the deprotonation fragments. ( a ) 1-D cut of potential energy curves of the considered states in the ionization and deprotonation: ground ( ) and first excited state ( A 1 Π u ) of the neutral molecule, the cation ground ( X 2 Π u ) and degenerate first excited state ( A 2 Π u ), and the dication ground ( ) and first excited state ( A 3 Π u ) along the anti-symmetric stretching coordinate R anti at R sym =0. The red vertical line indicates the tunnelling ionization and the grey curved line marks the second ionization step by electron recollision. ( b ) Density plot of the acetylene dication longitudinal recoil momentum as a function of the experimental CEP, φ , for 4 fs pulses at an intensity of 2 × 10 14 W cm −2 . CEP-integrated momenta are shown in the right panel. The dashed (dotted) lines shown correspond to CEP’s with maximum positive (negative) asymmetry in the ion emission, respectively. ( c ) Density plot for the asymmetry parameter, A ( p || ,φ), for C 2 H 2 2+ ions. ( d ) Density plot of the vector momentum sum of the recoil of the two (H + ,C 2 H + ) deprotonation fragments. ( e ) Density plot of the asymmetry parameter for the momentum sum of the deprotonation fragments (H + ,C 2 H + ). Full size image To confirm the population scenario of the dication, which involves ionization by the laser field followed by subsequent recollisional ionization and excitation ( Fig. 1a ), high-resolution spectra of the longitudinal (along the laser polarization axis) momentum p || for the doubly charged C 2 H 2 2+ recoil ions as a function of the CEP for 4-fs laser pulses at a peak intensity of 2 × 10 14 W cm −2 were recorded and are shown in Fig. 1b . Clear modulation of the dication’s momentum with the CEP is visible. To enhance the visibility of CEP-effects, it is useful to define an asymmetry parameter, A ( p || , φ ), as with N pos ( p || , φ ) and N neg ( p || , φ ) representing the yields for positive and negative momentum components p || , respectively. The 2-dimensional map in Fig. 1c for the dication shows high-amplitude asymmetry. Corroborated by previous studies on atoms [25] and diatomic molecules [26] , the dependence of the recoil-ion momentum on the CEP indicates that the doubly charged ion, at this laser intensity, is formed via an electron recollision process. Here, the free electron created in the first tunnelling event is guided by the laser field, and, for certain CEPs, the electron will return with sufficient energy to ionize the C 2 H 2 + ion. Because of momentum conservation during ionization, the momentum sum of the two ionized electrons is equal and opposite to the measured recoil momentum of the C 2 H 2 2+ ion (neglecting the small momentum contribution of the absorbed photons). The data in Fig. 1b,c indicate that—for the near-single cycle pulses used in the experiment—the electron recollision and the corresponding double ionization and excitation of C 2 H 2 2+ are controlled by the light waveform. This is analogous to previous findings on the non-sequential double ionization of argon with 4-fs pulses [25] , where it was shown that electron recollision can be limited to a single event by using sufficiently short, CEP-controlled laser pulses. Exploiting the applied coincident multi-particle detection scheme, the deprotonation channel has been identified by the coincidence of the H + and C 2 H + fragments following the dissociation of the dication. We can investigate the dependence of their yield on the CEP. Figure 1d,e shows the CEP-dependent momentum sum, p sum , of the coincident H + and C 2 H + fragments parallel to the laser field and the asymmetry that is derived from these data. A clear CEP dependence is visible in Fig. 1d,e exhibiting the same oscillatory behaviour as seen for the dication. The similarity of the two plots indicates that the recollision process is responsible for the recoil momentum of both the dication and the centre of mass motion of the reaction products after deprotonation. Directional laser-waveform control of the deprotonation As a signature of the deprotonation we investigate H + fragments from coincident creation of H + and C 2 H + upon the break-up of the dication. 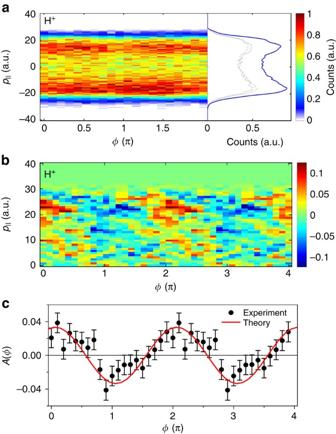Figure 2: Subfemtosecond directional control of deprotonation. (a) Density plot of the momentum of H+fragments as a function of CEP. CEP-integrated momenta are shown in the right panel. The dashed (dotted) lines shown correspond to CEP with maximum positive (negative) asymmetry in the ion emission, respectively. (b) Density plot for the asymmetry parameter,A(p||,φ), for the H+fragments. (c) The asymmetry parameter,A(φ), integrated over all momenta for H+ions. The error bars were derived via error propagation using the s.d. in the ion yields with positive and negative momenta. The clear oscillation in the asymmetry for the directional emission of H+fragments as a function of CEP under the given laser conditions demonstrates the CEP-control of the hydrogen emission direction. Also shown is the calculated asymmetry (solid red line) obtained from our quantum dynamical calculations (see text for details), which has been shifted in absolute CEP for best overlap with the experimental data since the absolute CEP is not known from the experiment. Figure 2a,b shows the momentum and asymmetry for H + ions. The directional control of the deprotonation reaction becomes visible when analysing the asymmetry of the H + emission, which is shown in Fig. 2b . Figure 2c shows the asymmetry parameter A ( φ ) that has been integrated over all momenta of the H + fragments. The observed preferential CEP-dependent ejection of protons to the left and right of the laser polarization axis illustrates the subfemtosecond steering of the hydrogen ejection. Figure 2: Subfemtosecond directional control of deprotonation. ( a ) Density plot of the momentum of H + fragments as a function of CEP. CEP-integrated momenta are shown in the right panel. The dashed (dotted) lines shown correspond to CEP with maximum positive (negative) asymmetry in the ion emission, respectively. ( b ) Density plot for the asymmetry parameter, A ( p || , φ ), for the H + fragments. ( c ) The asymmetry parameter, A ( φ ), integrated over all momenta for H + ions. The error bars were derived via error propagation using the s.d. in the ion yields with positive and negative momenta. The clear oscillation in the asymmetry for the directional emission of H + fragments as a function of CEP under the given laser conditions demonstrates the CEP-control of the hydrogen emission direction. Also shown is the calculated asymmetry (solid red line) obtained from our quantum dynamical calculations (see text for details), which has been shifted in absolute CEP for best overlap with the experimental data since the absolute CEP is not known from the experiment. Full size image To account for the asymmetric deprotonation, the well-known Tannor-Rice control scheme exploiting excited state dynamics [27] might appear to be a first candidate. However, for the current case, where the involved electronic state potentials are symmetric with respect to the deprotonation direction, an additional asymmetry has to be introduced by the laser field. We have performed quantum dynamical calculations to model the relevant molecular dynamics. The details of our calculations are given in the Methods section. The deprotonation of the dication is described in the basis of the symmetric |0 m > and anti-symmetric C-H stretching | n 0> modes with m , n being the number of vibrational quanta, and |0 m > and | n 0> implicitly including the respective time evolution factor . Around the minimum of PES, these modes correspond to the normal modes and their respective overtones. A linear combination of these modes, , will induce a wave packet motion along either one of the C-H stretching coordinates. When such a wave packet experiences a repulsive potential either the deprotonation of the left or the right H-atom is initiated. Two-dimensional (2D) PES along the normal mode coordinates ( R sym , R anti ) are calculated for the neutral, cationic, dicationic ground and excited states. The first excited state, the A 3 Π u state, of the dication turns out to be the important state for the reaction (see Fig. 1a and Methods section) and its 2D surface is shown in Fig. 3 . 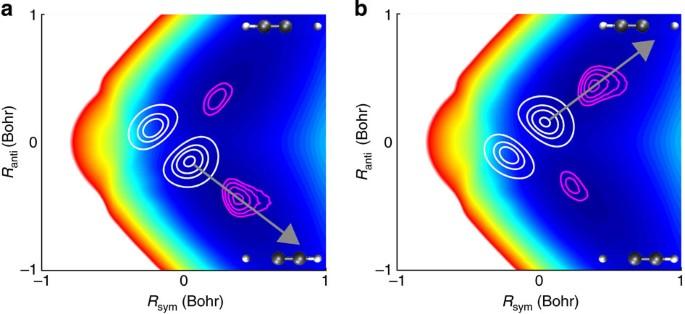Figure 3: The relevant first excited state of the dication for deprotonation. The state (A3Πu) is shown as a 2D-surface plotted against the symmetric and anti-symmetric stretching coordinates. The arrows inaandbindicate the two directions, into which protons can be emitted. To illustrate the control process, we plotted two wave packets representing the ideal superposition of(a) and(b). The initial wave packets are shown by white topographic lines, a snapshot of the same wave packet after 2.4 fs in magenta. The negative superposition (a) yields dominant cleavage of the left C-H bond, while the positive superposition (b) yields dominant cleavage of the right C-H bond. Figure 3: The relevant first excited state of the dication for deprotonation. The state ( A 3 Π u ) is shown as a 2D-surface plotted against the symmetric and anti-symmetric stretching coordinates. The arrows in a and b indicate the two directions, into which protons can be emitted. To illustrate the control process, we plotted two wave packets representing the ideal superposition of ( a ) and ( b ). The initial wave packets are shown by white topographic lines, a snapshot of the same wave packet after 2.4 fs in magenta. The negative superposition ( a ) yields dominant cleavage of the left C-H bond, while the positive superposition ( b ) yields dominant cleavage of the right C-H bond. Full size image From the stretching modes, only the anti-symmetric mode |10> is IR-active, and the incident light field is not resonant with the vibrational transitions. To prepare the required superposition, it is sufficient to address and control only the anti-symmetric |10> mode, via IR transitions. For the given light field, this happens in the neutral and cation. The symmetric mode contributions in the vibrational wave packet occur solely due to the ionization steps. The time-dependent population of the anti-symmetric mode |10> follows the electric field evolution of the few-cycle pulse (see Methods section). The CEP of the pulse imprints a certain phase ( ϕ CEP ) on the addressed anti-symmetric mode . When the few-cycle pulse is able to modify the phase of the anti-symmetric stretching mode, the sign in the superposition of the symmetric and anti-symmetric modes can be varied with the CEP and exhibits a modulation with a periodicity of 2π. To mimic the effect of the second ionization including the recolliding electron, the cationic wave packet is projected onto the dication. During the second ionization step, the intensity of the remaining light field is too low to significantly enhance the control of the asymmetric stretching mode |10> components. The main role of the recolliding electron is to provide the energy that is sufficient to reach the excited triplet state A 3 Π u . The energy of the recolliding electron can be evaluated for the given laser parameters to about 33 eV, corresponding to 3.17 U p [28] with the ponderomotive potential U p = I /(4 ω 2 ) (in atomic units) that depends on the laser intensity I and the angular frequency ω . An electron energy of 25 eV is enough to reach the A 3 Π u state of the dication. Because of the significant differences in the potential shape of the dicationic A 3 Π u state and the cationic ground state ( Fig. 1a ), higher vibrational quanta (| n 0> and |0 m >) up to the dissociation limit become now the dominant components of the vibrational wave packet and dissociation of the C-H bond can occur [13] . The preparation of the CEP-dependent features in the vibrational wave packet takes place in the neutral and cation, and is transferred to the dication in the second ionization. We observe that the propagation of the vibrational wave packet in the dication to either one of the dissociative channels (H + +CCH + and HCC + +H + , see Fig. 3 ) can be manipulated by the CEP. Evaluation of the fraction of the wave packet correlating with the individual dissociation channels provides the theoretical asymmetry plotted in Fig. 2c . The theoretical curve shows excellent agreement with the experimental data, which lends support to the described novel subfemtosecond control mechanism. The presented experimental and theoretical data support a new and very general coherent-control scheme, where the direction of proton ejection in a symmetric hydrocarbon is steered through manipulating the phases of the individual components of the vibrational wave packet. The CEP control-induced mechanism is substantially different from all previous studies, where electronic wave packets dominated the outcomes of the molecular dynamics [16] , in the context of which the enhancement of the asymmetry through selection of vibrational states has been reported [29] , [30] . While in the current proof-of-principle experiment, the degree of control was rather limited, it can be enhanced by using near-single cycle waveforms that are resonant with the optically active mode. With the advent and current development towards the generation of ultrashort, phase-stable light pulses in the mid-infrared [31] , substantial improvement of control is within reach. We expect the control scheme to be widely applicable to a variety of chemical processes, where the reactions of not only asymmetric but also symmetric molecules can be manipulated. Experimental set-up Linearly polarized laser pulses with a central wavelength of 750 nm, an energy of 150 μJ and a full width at half maximum of the temporal intensity envelope of 4 fs are generated at a repetition rate of 10 kHz in an amplified laser system. The laser intensity was kept stable on the level of 10%. The CEP of each laser pulse was recorded by sending a fraction of the laser beam (20 μJ) into a single-shot stereographic above-threshold ionization (Stereo-ATI) phase meter [32] . A detailed description of the CEP measurement and CEP tagging techniques can be found in ref. 33 . In brief, the time-of-flight spectra of electrons emitted along both directions of the laser polarization axis are recorded on either side of the apparatus. For each laser shot, the CEP is inferred from the asymmetry between the left and the right TOF spectra. Note that the CEP is measured up to a constant offset in the phase meter. In a recent study, we showed that slow drifts of the laser intensity can markedly affect the results of phase-tagged ionization yield measurements with long acquisition time [34] . To correct for any effects of small drifts of the laser parameters on the CEP measurement, we have applied the procedure outlined in ref. 34 , which had been tested to give reliable phase-tagged ion yields for the non-sequential double ionization of argon. The uncertainty in determining the CEP was on the order of 300 mrad during the entire measurement. A fraction (up to 15 μJ) of the remaining part of the laser beam is focused with a spherical mirror ( f =25 cm) into a well-localized (1 mm width) and cold supersonic gas jet of acetylene molecules in the centre of a REMI. Ions and electrons created in the laser focus (40 μm diameter) can be extracted by an electric field towards time- and position-sensitive MCP detectors at the left and right side of the instrument, respectively. In the current experiments, only ion signals were recorded. The ions’ impact positions were determined utilizing a two-dimensional delay line anode mounted behind the MCP. Pulses from the ends of the x and y delay lines and a time signal from the microchannel plate were registered by a multi-hit time-to-digital converter and recorded in event mode. From these data, off-line analysis provided the 3D vector momentum of each ionic fragment at the instant of double ionization. The deprotonation fragments are identified and isolated from other fragments by applying tight momentum sum conditions using the coincidence high-resolution PIPICO (Photo-Ion Photo-Ion) spectra [7] . Statistical evaluation of the asymmetry data To assess the statistical significance of the observed asymmetry, the data were subjected to a statistical test. Asymmetry curves were generated from the data for 1,000 different random re-orderings of the simultaneously recorded CEP values, that is, the CEP measured for an event was randomly associated with a different event before calculating the asymmetry. Any re-ordering should destroy the correlation of the data with the CEP, and those data can therefore be regarded as providing an upper limit for the noise of the measurement. The amplitude of the asymmetry oscillation was extracted from each test curve by a sinusoidal fit of the resulting asymmetry curve and plotted against the R 2 value in Fig. 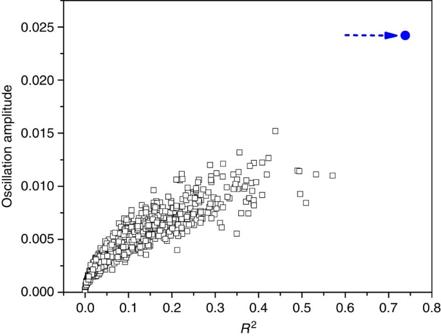Figure 4: Statistical evaluation of the asymmetry. In the measured data, the CEPs were randomized and the resulting asymmetry curve was fitted by a sinusoidal to extract the amplitude. This was repeated 1,000 times and the fitted amplitudes andR2values (see text) for each are plotted. The true experimental data are displayed as a blue point indicated by an arrow, demonstrating the statistical significance of the observed CEP-dependence. 4 , which is defined as: Figure 4: Statistical evaluation of the asymmetry. In the measured data, the CEPs were randomized and the resulting asymmetry curve was fitted by a sinusoidal to extract the amplitude. This was repeated 1,000 times and the fitted amplitudes and R 2 values (see text) for each are plotted. The true experimental data are displayed as a blue point indicated by an arrow, demonstrating the statistical significance of the observed CEP-dependence. Full size image where denotes the mean value of the asymmetry over all bins and f ( φ i ) the fitted asymmetry for bin i . The point corresponding to the true experimental data (non-randomized CEP ordering) is displayed as a blue point indicated by an arrow. It can be seen that this point shows a significantly larger goodness of the fit compared with the randomized test data. Therefore, despite its small amplitude, we conclude that the observed directional emission of protons is statistically significant. Quantum chemistry methods PES for ground and excited states of the neutral, cation and dication states of acetylene were calculated on the CASSCF[10,10], [9,10] and [8,10] level of theory, respectively, using the program package MOLPRO [35] with the 6-311++G** basis set as well as the dipole moments and transition dipole moments. Two-dimensional PES were calculated along the symmetric and anti-symmetric stretching coordinate with a step size of 0.05 a.u.. The PES were interpolated to 256 × 256 points for the evaluation of the vibrational eigenstates and the propagation of the vibrational wave packets. In the neutral molecule, only the IR-transitions play a role since the first excited state is separated by 7.8 eV (vertically) or 6.2 eV (adiabatically) and does not influence the ground state wave packet. Wave packet propagation The Chebychev propagator was used to solve the time-dependent Schrödinger equation. The time-dependent Schrödinger equation for the neutral molecule under the influence of the light field reads: with H n the Hamiltonian of , μ nn the associated dipole moment and ε ( t ) the near-single cycle laser field. The light field ε ( t ) was included in the dipole approximation: and was characterized by a full width at half maximum of 4 fs with a cycle-averaged intensity of 2 × 10 14 W cm −2 . The light field was discretized with a time step of 0.024 fs. The part of the laser interaction experienced by the neutral molecule has a duration of 4.8 fs (200 time steps) in correspondence to the time when the intensity maximum is reached and the system is ionized. During that period, the initial superposition is formed. All ionization steps are approximated by setting the vibrational wave packet onto the corresponding ionic state. In the first ionization step, the vibrational wave packet of the neutral molecule is transferred to the lowest cation states. The first two electronic states ( X 2 Π u and A 2 Π u ) in the cation are nearly degenerate and we assume an equal distribution over both states in the ionization of the neutral molecule. A second type of interaction with the laser field via electronic transitions back and forth between the states is possible and included for completeness in the total Hamiltonian given below. However, the transition dipole moment between those states is almost non-existent along the deprotonation modes and its effect is negligible. The time-dependent Schrödinger equation for the cation reads: with H 1 , H 2 the Hamiltonians of X 2 Π u , A 2 Π u of the cation, μ 11 , μ 22 the associated dipole moments, and μ 12 the almost zero transition dipole moment. The dissociation of the wave packet in the excited triplet state A 3 Π u of the dication was propagated for 480 fs with time steps of 0.24 fs. The part of the wave packet leaving the PES ( Fig. 3 ) on the top/bottom corresponds to the right/left deprotonation. Its amount is quantified by summing up all parts during the propagation Mechanism of the CEP control The neutral molecule experiences the part of the light field from time t 0 to t 1 (see Fig. 5a ). The population of, for example, the anti-symmetric mode |10> ( Fig. 5b ) follows the electric field of the few-cycle pulse. The CEP of the few-cycle pulse imprints a certain phase ( ϕ CEP ) on the eigenfunction of , which leads through superposition with the |01> mode (populated in the ionization) to the directional deprotonation. Ionization is assumed to happen at maximal field strength (see blue line at t 1 in Fig. 5b ). From the evolution of the |10> population, it becomes obvious that the ionization step is crucial to populate the |10> mode as the interaction with the complete non-resonant light field would induce neither population (shown in red) nor phase information transfer. The first ionization transfers the vibrational wave packet to the cation. The major part of the wave packet is still the |00> component with no directional preference. However, because of the slight difference in the shape of the neutral and cationic potential energy curves now also the IR inactive mode |01> is slightly populated with a system dependent, but uncontrollable phase . The population of the IR-active mode |10> is further increased by the interactions with the remaining light field ( Fig. 5b , green line) and the imprinted phase in the superposition, defining the direction of the wave packet oscillation, is strengthened. The cation experiences the part of the light field from time t 1 to t 2 ( Fig. 5a ). Contributions from higher vibrational quantum numbers may occur, but play a minor role. The prepared wave packet retains the memory of direction, when transferred to the dication in the final step. 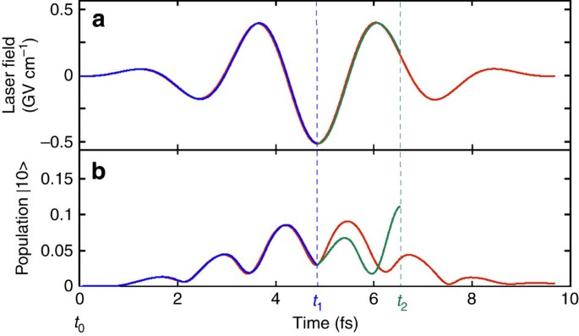Figure 5: Laser-field control of asymmetric hydrogen bond breaking. (a) Electric field waveform of the near-single-cycle laser pulse used in the calculations (red line). The parts of the field that act on the neutral and cation are displayed as blue and green lines, respectively. (b) Population of the IR-active mode |10>. The population induced in the neutral molecule is shown as blue line. At the peak of the laser field (t1), the |10> population is transferred to the cation and its evolution is shown as the green line. Recollisional excitation, 1.7 fs (t2) later, transfers the population to theA3Πustate of the dication, from where dissociation can occur. Now the eigenfunctions constituting the vibrational wave packet are continuum wavefunctions. Without ionization, interaction with the entire field would induce only a transient population shown as red line, which vanishes with the end of the laser pulse. Figure 5: Laser-field control of asymmetric hydrogen bond breaking. ( a ) Electric field waveform of the near-single-cycle laser pulse used in the calculations (red line). The parts of the field that act on the neutral and cation are displayed as blue and green lines, respectively. ( b ) Population of the IR-active mode |10>. The population induced in the neutral molecule is shown as blue line. At the peak of the laser field ( t 1 ), the |10> population is transferred to the cation and its evolution is shown as the green line. Recollisional excitation, 1.7 fs ( t 2 ) later, transfers the population to the A 3 Π u state of the dication, from where dissociation can occur. Now the eigenfunctions constituting the vibrational wave packet are continuum wavefunctions. Without ionization, interaction with the entire field would induce only a transient population shown as red line, which vanishes with the end of the laser pulse. Full size image How to cite this article: Alnaser, A. S. et al. Subfemtosecond steering of hydrocarbon deprotonation through superposition of vibrational modes. Nat. Commun. 5:3800 doi: 10.1038/ncomms4800 (2014).